Image transport through a disordered optical fibre mediated by transverse Anderson localization Transverse Anderson localization of light allows localized optical-beam-transport through a transversely disordered and longitudinally invariant medium. Its successful implementation in disordered optical fibres recently resulted in the propagation of localized beams of radii comparable to that of conventional optical fibres. Here we demonstrate optical image transport using transverse Anderson localization of light. The image transport quality obtained in the polymer disordered optical fibre is comparable to or better than some of the best commercially available multicore image fibres with less pixelation and higher contrast. It is argued that considerable improvement in image transport quality can be obtained in a disordered fibre made from a glass matrix with near wavelength-size randomly distributed air-holes with an air-hole fill-fraction of 50%. Our results open the way to device-level implementation of the transverse Anderson localization of light with potential applications in biological and medical imaging. Anderson localization is the absence of diffusive wave propagation in certain disordered media [1] , [2] , [3] , [4] . Transverse Anderson localization was first introduced by Abdullaev et al. [5] and De Raedt et al. [6] In the treatment suggested by De Raedt et al. , an optical wave system is studied in which the refractive index profile is random in the transverse plane and is invariant in the longitudinal direction. An optical beam launched in the longitudinal direction can become localized in the transverse plane due to the strong random scattering from the transverse random index fluctuations and can propagate in the longitudinal direction with a finite beam radius, similar to a conventional optical fibre. The radius of the localized beam depends on the extent of the fluctuations in the value of the refractive index, the characteristic length over which the fluctuations occur, as well as the wavelength of the light [7] , [8] , [9] . Transverse Anderson localization was first observed experimentally in 2007 (ref. 10 ). That experiment, carried out in a photo-refractive crystal, utilized refractive index variations of the order of 10 −4 . Such small variations in the refractive index of random sites result in a very large mean value and s.d. of the localized beam radius [9] . For device applications that benefit from the waveguiding properties of transverse Anderson localization, the mean localized beam radius should be comparable to or smaller than that of conventional optical fibres and large sample-to-sample variations in the beam radius are not acceptable. Therefore, it is necessary to increase the refractive index difference of the random sites. We recently demonstrated transverse Anderson localization of light in a polymer random optical fibre medium with refractive index fluctuations of order 0.1 (ref. 7 ). The polymer Anderson localized fibre (p-ALOF) allowed for the simultaneous propagation of multiple beams in a single strand of disordered optical fibre [8] with potential applications in beam-multiplexed optical communications and optical imaging. Here we demonstrate optical image transport using transverse Anderson localization of light, specifically in a disordered optical fibre. The possibility of using disordered optical fibre for some form of image transport was expected, given the earlier demonstration of spatial beam multiplexing in p-ALOF (ref. 8 ). The novelty of the presented work is in demonstrating that the image transport quality can be of a comparable or higher quality than the commercially available multicore imaging optical fibres. It is remarkable that the high quality image transport is achieved because of, not in spite of, the high level of disorder and randomness in the imaging system. Image transport in disordered fibres Multicore optical fibres have been used extensively in high-resolution optical imaging [11] ; however, the transmitted images are inherently pixelated due to the discrete nature of the light-guiding array of cores, and the inter-core coupling can reduce the image contrast and result in blurring [12] , [13] . Certain structural non-uniformities such as variations in the size of the cores were shown by ref. 14 to improve the image transport quality. A weakly disordered fibre array was also studied in ref. 15 and was shown to induce diffusive spreading or localization at a few sites across the fibre. High numerical aperture guiding cores were also suggested by ref. 13 to reduce core-to-core coupling and blurring in imaging applications. A highly disordered optical fibre with large refractive index fluctuations can transport high quality images, as it provides a high degree of structural non-uniformity as well as a sufficiently large local numerical aperture. More rigorously, the image transport quality is due to the transverse Anderson localization phenomenon that creates localized transport channels with finite radii (localized optical modes) through the disordered imaging waveguide [16] , [17] . A higher amount of disorder and a larger level of fluctuation in the refractive index provides stronger beam localization, hence improving the image resolution. It is also responsible for the reduction in the value of the s.d. in the localized beam radius as a consequence of the self-averaging behaviour [7] , [18] , [19] , ensuring uniform image transport quality across the fibre facet. The coherent transverse coupling and blurring is considerably reduced, because the transverse disorder results in strong spatial incoherence across the beam, akin to using incoherent light to eliminate speckles in an imaging system. Therefore, even a laser can be readily used for illumination in this image fibre to obtain a higher signal-to-noise ratio, without worrying about its undesirably high spatial coherence. Image transport in p-ALOF The fabrication of the p-ALOF used in these imaging experiments is described in detail in (refs 7 , 20 ); In brief, it is composed of 40,000 strands of poly methyl methacrylate (PMMA) and 40,000 strands of poly styrene (PS) drawn to a square profile with a side width of 250-μm and site sizes of about 0.9-μm (see Methods). A magnified scanning electron microscope (SEM) image of a portion of the tip of the p-ALOF is shown in Fig. 1a , where the PMMA sites (refractive index of 1.49) are darker compared with the lighter PS sites (refractive index of 1.59). Also shown in Fig. 1b , for comparison, is an SEM image of a portion of the tip of a glass disordered fibre earlier reported in ref. 21 , where the darker sites are the airholes. In the following, we demonstrate high-quality optical image transport through the p-ALOF related to Fig. 1a mediated by transverse Anderson localization of light. We also argue that a higher disorder density is required for quality image transport through the glass disordered fibre of Fig. 1b and a higher air-hole fill-fraction of nearly 50% should result in a very high-quality image fibre. 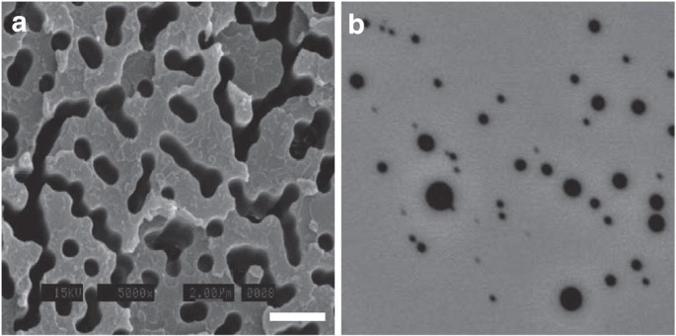Figure 1: SEM images of the disordered fibres. Magnified SEM image of a portion of the tip of the (a) p-ALOF and (b) glass-disordered fibre. For p-ALOF in (a), the PMMA (PS) sites are darker (lighter) in colour. For the glass-disordered fibre, the darker sites are the airholes. Scale bar=4 μm. Figure 1: SEM images of the disordered fibres. Magnified SEM image of a portion of the tip of the ( a ) p-ALOF and ( b ) glass-disordered fibre. For p-ALOF in ( a ), the PMMA (PS) sites are darker (lighter) in colour. For the glass-disordered fibre, the darker sites are the airholes. Scale bar=4 μm. Full size image To investigate the image transport capability of the p-ALOF, optical images of the ‘numbers’ from group 3 and group 4 on an 1951 U.S. Air Force resolution test chart (1951-AFTT), Fig. 2 , are launched using a 405 nm laser diode into the p-AOLF (see Methods). Different numbers in each group are of the same size. The transported images for the groups 3 and 4 are shown in Figs 3 and 4 , respectively, after 5 cm of propagation in the p-ALOF. Theoretically, the minimum resolution of the images is determined by the width of the point spread function of the p-ALOF imaging setup, which is comparable to the localization length. The transverse localization length (localized beam radius) of the p-ALOF at 405 nm wavelength was calculated to be smaller than 10 μm (ref. 9 ). In practice, the imaging resolution in p-ALOF is limited by the quality of the cleaving and polishing of the p-ALOF surface. The fibre surface quality both at the input and output is partially responsible for the distortions observed in the transported images in Figs 3 and 4 . 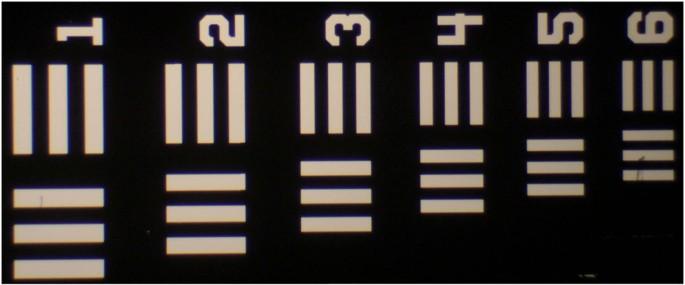Figure 2: 1951 U.S. Air Force test target. Elements of a group on the 1951-AFTT. Figure 2: 1951 U.S. Air Force test target. Elements of a group on the 1951-AFTT. 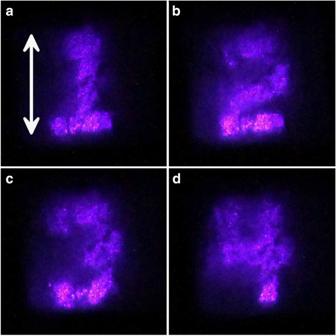Figure 3: Transported images through the disordered fibre. Transported images of different numbers through 5 cm of p-ALOF, (a–d), related to the group 3 on the 1951-AFTT (experimental measurements). Scale bar=120 μm. Full size image Figure 3: Transported images through the disordered fibre. Transported images of different numbers through 5 cm of p-ALOF, ( a – d ), related to the group 3 on the 1951-AFTT (experimental measurements). Scale bar=120 μm. 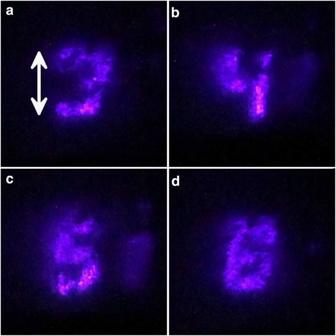Figure 4: Transported images through the disordered fibre. Transported images of the numbers through 5 cm of p-ALOF, (a–d), related to the group 4 on the 1951-AFTT (experimental measurements). Scale bar=60 μm. Full size image Figure 4: Transported images through the disordered fibre. Transported images of the numbers through 5 cm of p-ALOF, ( a – d ), related to the group 4 on the 1951-AFTT (experimental measurements). Scale bar=60 μm. Full size image Comparison with commercial multicore image fibres The imaging performance of the p-ALOF compares with some of the best commercially available multicore imaging optical fibres, as shown in Fig. 5 . The transported images over 5 cm of the number ‘6’ from group 5 of the 1951-AFTT test chart are compared between p-ALOF in Fig. 5a , Fujikura FIGH-10-350S in Fig. 5b and Fujikura FIGH-10-500N in Fig. 5c . The visual image quality of the transported image through the p-ALOF is clearly better than FIGH-10-350S and is comparable to FIGH-10-500N. We would like to emphasize that the feature sizes in Fig. 5 are of the order of 10–20 μm. The Rayleigh range for this level of resolution and the 405 nm laser wavelength is approximately 0.8–3 mm, which is substantially shorter than the 5 cm propagation length in these image fibres. Therefore, the imaging results are non-trivial and cannot be obtained using bulk propagation or conventional multimode optical fibres. To quantify the perceived image quality of the transported images, we use the mean structural similarity index (MSSIM) throughout this manuscript. Details and justifications on the use of this metric are given in the Methods section. The MSSIM values are 0.5877 for Fig. 5a , 0.5501 for Fig. 5b and 0.5591 for Fig. 5c . 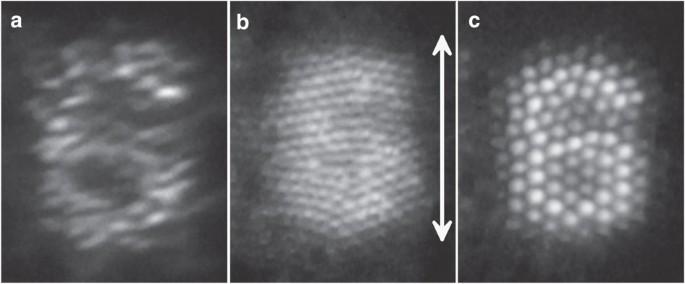Figure 5: Transported images through the disordered fibre and the commercial image fibres. Transported images related to group 5 of the 1951-AFTT test chart in (a) p-ALOF, (b) FIGH-10-350S image fibre and (c) FIGH-10-500N image fibre (experimental measurements). Scale bar in (b) is 30 μm-long and the same scale bar can be used for (a) and (c). Each fibre is approximately 5 cm long. The MSSIM image quality values for the images are (a) 0.5877, (b) 0.5501 and (c) 0.5591. Figure 5: Transported images through the disordered fibre and the commercial image fibres. Transported images related to group 5 of the 1951-AFTT test chart in ( a ) p-ALOF, ( b ) FIGH-10-350S image fibre and ( c ) FIGH-10-500N image fibre (experimental measurements). Scale bar in ( b ) is 30 μm-long and the same scale bar can be used for ( a ) and ( c ). Each fibre is approximately 5 cm long. The MSSIM image quality values for the images are ( a ) 0.5877, ( b ) 0.5501 and ( c ) 0.5591. Full size image Using the optical and physical parameters of the p-ALOF, Fujikura FIGH-10-350S and Fujikura FIGH-10-500N, we repeat the experiment of Fig. 5 using the numerical simulation and show the results in Fig. 6a–c . The numerical simulation is detailed in the Methods section. Similar to Fig. 5 , the transported images are over 5 cm of the number ‘6’ created using the GIMP image editor and nearly the same size as the group 5 of the 1951-AFTT test chart and are compared between p-ALOF in Fig. 6a , Fujikura FIGH-10-350S in Fig. 6b and Fujikura FIGH-10-500N in Fig. 6c . 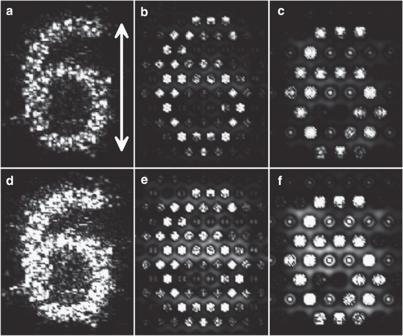Figure 6: Simulation of image transport through the disordered fibre and the commercial image fibres. Transported images related to group 5 of the 1951-AFTT test chart in (a) p-ALOF, (b) FIGH-10-350S image fibre and (c) FIGH-10-500N image fibre (numerical simulations). The scale bar in (a) is 30 μm long and the same scale bar can be used for other subfigures. Each fibre is approximately 5 cm long. The top row (subfigures (a), (b) and (c)) can be compared with the experimental results shown inFig. 5. Subfigures (d), (e) and (f) in the bottom row are the same as subfigures (a), (b) and (c) in the top row, except the images are saturated by changing the colour axis in grey-scale colormap in Matlab. The colour axis of [0,1] in subfigures (a), (b) and (c) is changed to colour axis of [0,0.3] in (d), (e) and (f). The MSSIM image quality values for the images are (a) 0.637, (b) 0.615 and (c) 0.6257. The MSSIM values for (d), (e) and (f) are the same as (a), (b) and (c), respectively. Figure 6: Simulation of image transport through the disordered fibre and the commercial image fibres. Transported images related to group 5 of the 1951-AFTT test chart in ( a ) p-ALOF, ( b ) FIGH-10-350S image fibre and ( c ) FIGH-10-500N image fibre (numerical simulations). The scale bar in ( a ) is 30 μm long and the same scale bar can be used for other subfigures. Each fibre is approximately 5 cm long. The top row (subfigures ( a ), ( b ) and ( c )) can be compared with the experimental results shown in Fig. 5 . Subfigures ( d ), ( e ) and ( f ) in the bottom row are the same as subfigures ( a ), ( b ) and ( c ) in the top row, except the images are saturated by changing the colour axis in grey-scale colormap in Matlab. The colour axis of [0,1] in subfigures ( a ), ( b ) and ( c ) is changed to colour axis of [0,0.3] in ( d ), ( e ) and ( f ). The MSSIM image quality values for the images are ( a ) 0.637, ( b ) 0.615 and ( c ) 0.6257. The MSSIM values for ( d ), ( e ) and ( f ) are the same as ( a ), ( b ) and ( c ), respectively. Full size image Similar to the experimental results of Fig. 5 , the numerical simulation shown in Fig. 6 indicates that the visual image quality of the transported image through the p-ALOF is better or comparable to the Fujikura image fibres. The experiment and numerics are in reasonable agreement, but there are differences, as well. Possible sources of difference can be traced back to uncertainties in relating the experiment to numerics. The MSSIM values are 0.637 for Fig. 6a , 0.615 for Fig. 6b and 0.6257 for Fig. 6c . Sources of systematic image degradation In the experiment, a good precision in the butt-coupling of the test target to the input fibre is needed to obtain high-quality output images. An important source of uncertainty is the surface quality of the fibres, determining the precision in coupling the input profile from the test target and coupling the output to the CCD camera. The Fujikura image fibres are cleaved and polished using commercial-grade equipment, while the p-ALOF is hand-cleaved and polished using the lapping paper from Thorlabs. These variations and uncertainties cannot be easily accounted for in the numerical simulation without extensive surface quality characterizations of p-ALOF and Fujikura image fibres and are likely not very illuminating, considering that the p-ALOF images can be improved if specialized equipment for cleaving and polishing polymer fibres are used to improve its surface quality. Another possible source of uncertainty is the degree of spatial coherence of the laser used to illuminate the test target. The spectral bandwidth of the laser also contributes the fuzziness of the experiment, while the single-frequency numerical simulation looks more pixelated. We note that the scalar wave equation has been benchmarked extensively with the full vectorial beam propagation method, and the results have shown to be in excellent agreement for the numerical apertures relevant in these simulations [9] . The quality of the imaging setup and the saturation of the CCD camera versus the saturation of the images generated using numerics can be another source of perceived difference between the experiment and numerics. The images of Fig. 6a–c are plotted using the colour axis of [0,1] in grey-scale colormap in Matlab. In Fig. 6d–f , the colour axis is changed to [0,0.3] for the same simulation, resulting in a more fuzzy image. It should also be noted that the numerical simulations are for images at the tip of the fibre, while those from the experiment are after passing through the near-field imaging setup discussed in the Methods. The simulated images of multicore image fibres in Fig. 6 look quite different from the experiment in Fig. 5 , even when one takes into account the uncertainties mentioned above. This issue was pointed out in ref. 14 , where it was suggested that the discrepancy between theory and experiment is because the image fibres are not composed of identical cores. The published core size specification is likely the average value with potentially a large s.d. While it is possible to build a concrete model to investigate this issue in detail, it is beyond the scope and interests of this manuscript. Localization is responsible for enhanced image transport The discussion so far has mainly focused on the perceived quality of the images in Figs 5 and 6 . Because the intention of this manuscript is to argue that transverse Anderson localization induced by the disorder results in a higher quality image transport when compared with multicore image fibres, it is important to ensure that similar specifications are used for the disordered and multicore image fibres to ensure that the comparison is conducted fairly. The core and cladding refractive indices of the Fujikura image fibres are 1.5 and 1.446, respectively, for which the index difference of 0.054 is lower than that of p-ALOF (0.1). To isolate the effect of disorder and Anderson localization on the image transport quality and eliminate the differences due to the numerical apertures, an image fibre with the same numerical aperture as p-ALOF and the structural parameters of FIGH-10-500N is modelled using the numerical simulation. The input image is the word ‘UWM,’ where each letter is 44-μm high, the lines in the letters are 6-μm thick and the letters are separated by 26-μm. The intensity profiles of the transported images at the wavelength of 405 nm after 5 cm of propagation in p-ALOF and the image fibre with a raised numerical aperture are compared in Fig. 7a,b . The quality of the transported image in Fig. 7a is higher than that of the modified image fibre in Fig. 7b . There is considerable pixelation in Fig. 7b and a low intensity halo of illuminated cores fills the area in between the main lines of the transported letters. It appears that even with the same level of index difference, p-ALOF provides a comparable or better quality image transport compared with the multicore image fibre. 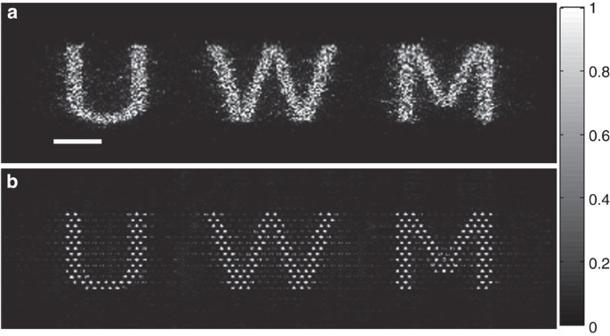Figure 7: Simulation of image transport through the disordered fibre and an image fibre. The intensity profile of the ‘UWM’ image after 5 cm of propagation and at the wavelength of 405 nm in a (a) p-ALOF, (b) modified image fibre with the refractive index difference of 0.1 between the cores and the clad, using numerical simulations. The scale bar in (a) is 20 μm long and the same scale bar can be used for (b). The MSSIM image quality value for the images are (a) 0.8923 and (b) 0.6263. Figure 7: Simulation of image transport through the disordered fibre and an image fibre. The intensity profile of the ‘UWM’ image after 5 cm of propagation and at the wavelength of 405 nm in a ( a ) p-ALOF, ( b ) modified image fibre with the refractive index difference of 0.1 between the cores and the clad, using numerical simulations. The scale bar in ( a ) is 20 μm long and the same scale bar can be used for ( b ). The MSSIM image quality value for the images are ( a ) 0.8923 and ( b ) 0.6263. Full size image It should be noted that the images in Fig. 7 appear to be of higher quality compared with Figs 5 and 6 , simply because they are of different sizes and resolutions. The MSSIM values are 0.8923 for Fig 7a and 0.6263 for Fig. 7b . As further concrete evidence that the disorder is responsible for the higher image transport quality, the quantitative MSSIM metric for image quality assessment is compared in Fig. 8 for a collection of multicore image fibres with and without disorder. The blue squares in Fig. 8 represent the value of MSSIM for image transport through 5 cm of disorder-free (Δ=0) periodic image fibre as a function of the periodicity Λ. The radius of each individual core is 1.45 μm, which is the same as the mean radius of the cores in the FIGH-10-500N imaging fibre. The refractive index difference between the cores and common cladding is 0.1. The image that is transported through the image fibre is the number ‘6’ created using the GIMP image editor and is 65 μm high. In the case of disorder-free periodic image fibre, MSSIM is low for small Λ as expected because of the enhanced core-to-core coupling. It is also low for large Λ due to the pixelation effect. In general, the optimum Λ for the highest value of MSSIM depends on the numerical aperture and the radius of the individual core. 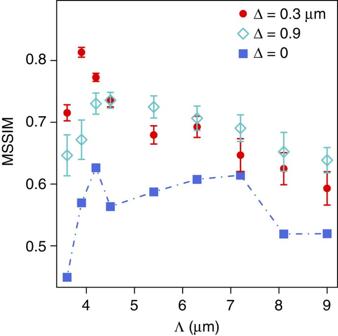Figure 8: Quantitative assessment of image transport quality through disordered fibres. The MSSIM metric for image quality assessment is compared for periodic image fibres as a function the core periodicity Λ. The blue squares represent disorder-free (Δ=0) periodic cores of radius 1.45 μm. The red circles and cyan diamonds represent disordered (Δ≠0) periodic cores of mean radius 1.45 μm with uniform random radius variations in the interval [−0.3 μm, 0.3 μm] and [−0.9 μm, 0.9 μm], respectively. The error bars signify one s.d. around the mean MSSIM obtained from thirty realizations of each case. Figure 8: Quantitative assessment of image transport quality through disordered fibres. The MSSIM metric for image quality assessment is compared for periodic image fibres as a function the core periodicity Λ. The blue squares represent disorder-free (Δ=0) periodic cores of radius 1.45 μm. The red circles and cyan diamonds represent disordered (Δ≠0) periodic cores of mean radius 1.45 μm with uniform random radius variations in the interval [−0.3 μm, 0.3 μm] and [−0.9 μm, 0.9 μm], respectively. The error bars signify one s.d. around the mean MSSIM obtained from thirty realizations of each case. Full size image The red circles and cyan diamonds in Fig. 8 represent the value of MSSIM for image transport through disordered (Δ≠0) image fibres. The radius of each individual core is chosen from a uniform distribution in the interval [1.45 μm−Δ, 1.45 μm+Δ]. Therefore, the mean radius is the same as that of the periodic case. Δ=0.3 μm for red circles and Δ=0.9 μm for cyan diamonds. For each image fibre, the value of MSSIM is calculated using the transported image. The numerical experiment is repeated 30 times for each representation of the disorder (at each Λ and Δ), to obtain sufficient statistics, where the error bars in MSSIM signify one s.d. around the mean MSSIM. It is observed that, at each value of Λ, the presence of the disorder improves the quality of the transported image. A detailed analysis shows that the maximum value of MSSIM is obtained for Λ=3.9 μm and Δ=0.3 μm. Although the disordered multicore image fibre explored in here differs from the structure of the p-ALOF, this numerical experiment provides further evidence in support of the claim that the presence of disorder can enhance the quality of the image transport. Further evidence on the effect of the disorder on improving the quality of image transport in multicore image fibre is provided in Supplementary Fig. 1 . In Supplementary Fig. 2 , the evolution of MSSIM with the propagation distance is compared between periodic and disordered multicore image fibres, as well as the p-ALOF. In all cases, the image quality drops in the first few millimeters of propagation and then saturates near the final value. The saturated MSSIM is considerably larger for the disordered fibres. Also, the MSSIM value for the p-ALOF is higher than the best disordered multicore image fibre with Δ=0.3 μm. This presents another concrete evidence that the p-ALOF is comparable or better than conventional multicore image fibres. We emphasize that the value of MSSIM depends on the size of the transported image and the MSSIM numbers reported in Supplementary Fig. 2 should only be compared with that of images with the same size. Impact of the wavelength on image quality For image transport through multicore imaging optical fibres, a longer optical wavelength increases the inter-core coupling strength and therefore lowers the quality of image transport. A similar effect can be observed in Anderson localized optical fibres as the mean localized beam radius has been shown to be larger for a longer wavelength [9] . In Fig. 9 , a longer wavelength of 633 nm is used for the numerical simulation of the image transport. The results must be compared with Fig. 6 . 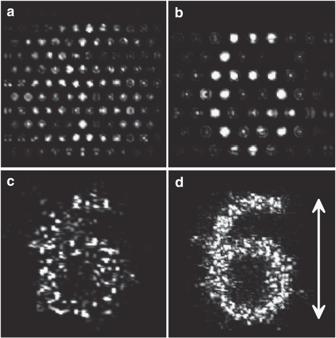Figure 9: Simulation of image transport at a longer wavelength of 633 nm. Numerical simulation of transported images related to group 5 of the 1951-AFTT test chart in (a) FIGH-10-350S image fibre, (b) FIGH-10-500N image fibre and (c) p-ALOF. Each fibre is approximately 5 cm long. The simulation wavelength is 633 nm and lower quality imaging is obtained, as expected, when compared withFig. 6at 405 nm wavelength. (d) is similar to (c), except an air-glass material with the index difference of 0.5 is assumed instead of 0.1 related to the polymer p-ALOF of (c). The scale bar in (d) is 20 μm long and the same scale bar can be used for (a), (b) and (c). The MSSIM image quality value for the images are (a) 0.3385, (b) 0.5396, (c) 0.6119 and (d) 0.6509. Figure 9 shows the numerical simulation of transported images related to group 5 of the 1951-AFTT test chart in (a) FIGH-10-350S image fibre, (b) FIGH-10-350S image fibre and (c) p-ALOF, using the 633 nm wavelength. The quality of the transported image at 633 nm is substantially lower than at 405 nm wavelength for all cases. For p-ALOF, the localization radius was calculated to be smaller than 10 μm at 405 nm wavelength and nearly 30 μm at 633 nm wavelength [9] . Because the localization radius determines the image transport resolution in a disordered optical fibre, the resolution is nearly three times lower at 633 nm than at 405 nm wavelength. For image fibres, longer wavelength results in a larger modal overlap between the cores, hence increasing core-to-core coupling and blurring of the image. It must be noted that the quality for imaging through the p-AOLF at the wavelength of 633 nm is still higher than that of the multicore image fibres at the same wavelength. The MSSIM values are 0.3385 for Fig. 9a , 0.5396 for Fig. 9b , 0.6119 for Fig. 9c and 0.6509 for Fig. 9d . Figure 9: Simulation of image transport at a longer wavelength of 633 nm. Numerical simulation of transported images related to group 5 of the 1951-AFTT test chart in ( a ) FIGH-10-350S image fibre, ( b ) FIGH-10-500N image fibre and ( c ) p-ALOF. Each fibre is approximately 5 cm long. The simulation wavelength is 633 nm and lower quality imaging is obtained, as expected, when compared with Fig. 6 at 405 nm wavelength. ( d ) is similar to ( c ), except an air-glass material with the index difference of 0.5 is assumed instead of 0.1 related to the polymer p-ALOF of ( c ). The scale bar in ( d ) is 20 μm long and the same scale bar can be used for ( a ), ( b ) and ( c ). The MSSIM image quality value for the images are ( a ) 0.3385, ( b ) 0.5396, ( c ) 0.6119 and ( d ) 0.6509. Full size image Impact of the disorder refractive index difference on image quality A higher value of the refractive index difference between the random sites in a disordered fibre such as p-ALOF is expected to improve the image transport quality by decreasing the localized beam radius [9] . An ideal disordered image fibre is made from a glass matrix with wavelength-size randomly distributed air-holes to provide a refractive index contrast of 0.5 between high- and low-index sites. The ideal air-hole fill-fraction is at 50% for maximum transverse scattering and minimum localized beam radius [9] . In Fig. 9d , we show the image transport through a disordered fibre with the same geometrical parameter of p-ALOF, but the refractive index values of the high- and low-index sites are set at 1.5 and 1.0, respectively, for the wavelength of the 633 nm. The quality of image transport in Fig. 9d is substantially better than Fig. 9c . We note that not only is the average localized beam radius lower in a properly designed glass-air disordered optical fibre compared with a p-ALOF, but there also are fewer sample-to-sample variations in the localized beam radius. Therefore, a higher image transport quality is expected with a more uniform performance across the fibre. Signal attenuation along the fibre Much lower intrinsic attenuation is expected in silica-based fibres compared with polymer fibres for longer image transport. In fact, 16 cm has been the longest p-ALOF sample that has been successfully used for imaging; transported images of the numbers ‘1’ and ‘6’ from group 3 of the 1951-AFTT test chart are shown in Fig. 10 . The maximum length for image transport in the p-ALOF is both a result of optical attenuation and the variations in the thickness of the optical fibre in the draw process. White light has been used for the image transport in Fig. 10 , and the output images appear red because the attenuation of the polymer materials used in p-ALOF is minimum for the red colour in the visible spectrum. The large variations in the thickness of the optical fibre in the draw process and the accumulated dust and humidity during the week-long stacking of the fibres due to the considerable static electrical charges that build up on the polymer fibres result in a loss of around 0.5 dB cm −1 at 633 nm. However, it is expected that by assembling the fibres in a clean-room environment and using a more stable draw process, the length of p-ALOF image fibres can be extended to at least several meters. 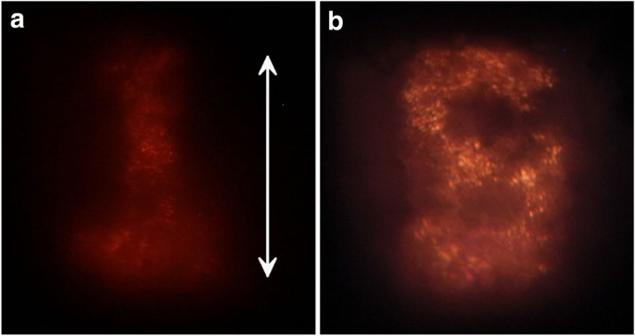Figure 10: Image transport through the disordered fibre over a longer distance. Transported images of the numbers ‘1’ and ‘6’ from group 3 of the 1951-AFTT test chart through a 16 cm-long p-ALOF sample are shown using a white light source (experimental measurements). The scale bar in (a) is 120 μm long and the same scale bar can be used for (b). Figure 10: Image transport through the disordered fibre over a longer distance. Transported images of the numbers ‘1’ and ‘6’ from group 3 of the 1951-AFTT test chart through a 16 cm-long p-ALOF sample are shown using a white light source (experimental measurements). The scale bar in ( a ) is 120 μm long and the same scale bar can be used for ( b ). Full size image A glass-air disordered optical fibre would be an ideal solution to the attenuation problem. Moreover, it is possible to obtain high quality fibre-end surfaces by using standard cleaving and polishing equipment in the laboratory. For the glass-air disordered fibres reported in ref. 21 and shown in Fig. 1b , transverse Anderson localization can be observed only near the boundary, because their air fill-fraction is 2–5% in the central regions, which is far below the ideal 50%; even near the boundary where transverse Anderson localization is observed, the localized beam radius is too large to be suitable for image transport. Comparison with other advanced fibre-based imaging methods Finally, it would be important to compare the advantages and disadvantages of imaging using the disordered optical fibres with other available fibre-based techniques. For example, Choi et al. [22] recently developed a highly interesting technique to use a single-core multimode optical fibre for endoscopic imaging. They relied on pre- and post-processing techniques to evaluate the transmission matrix of a multimode optical fibre to address the modal dispersion. Also, speckle imaging and turbid lens imaging methods are used to eliminate distortions. The post-processing limits the image acquisition time to one frame per second. In comparison, the disordered fibre provides a one-to-one map between the object and image plane, and no additional optics or pre- and post-processing is required to obtain the image. Therefore, image acquisition time is negligible. Another advantage of the disordered fibre-imaging over the technique presented by Choi et al. [22] is that their method does not support a fully flexible endoscopic operation due to the variation of the transmission matrix induced by the bending and twisting of the fibre. The beam localization in disordered fibre is very robust, even in very tight bends as shown in ref. 8 , so it can easily operate in a fully flexible endoscopic system. The main advantage of the method of ref. 22 over the disordered fibre-imaging is the imaging resolution. They report 12,300 effective image pixels over the 200 μm diameter core of the fibre, hence a pixel size of 6.4 λ 2 . On the basis of our simulations, even the best glass-air disordered fibres can only achieve pixel resolution of larger than 30 λ 2 , which is lower than that reported by Choi et al. In contrast, the disordered fibre is easily scalable, so it is conceivable the fabricate disordered fibres with millimeter-size cross-sections for ultra-wide-area and nearly instantaneous imaging for streaming videos, while the post-processing would make other techniques prohibitively slow. It must also be noted that the disordered fibre is inherently a multimode fibre, and the technique employed by Choi et al. can be applied to the disordered fibre as well. In that case, the localized nature of the beam transport and also the direct knowledge of transported images, albeit at a slightly lower resolution, can potentially reduce the post-processing time in their technique. The image transport quality is comparable to or better than some of the best commercially available multicore image fibres with less pixelation and higher contrast. In practice, the imaging resolution in p-ALOF is limited by the quality of the cleaving and polishing of the p-ALOF surface, and the maximum transport distance is limited by the optical attenuation as well as the variations in the thickness of p-ALOF in the draw process. The ultimate disordered image fibre will be made from a glass matrix with wavelength-size randomly distributed air-holes with an air-hole fill-fraction of 50%. The low optical attenuation in glass-air material is essential for transporting images over longer distances than reported here. The large index difference between the glass matrix and the air-holes and 50% air-hole fill-fraction provides maximum scattering in the transverse plane to reduce the localization beam radius and to minimize the width of the imaging point spread function. The large transverse scattering is also responsible for reducing the beam-to-beam variation of the localization radius. A small value of the s.d. is essential for device applications, as one expects to observe a nearly uniform width of the point spread function across the tip of the image fibre as well as among fibre samples. The reduction in the value of the s.d. of the localized beam radius is due to the self-averaging behaviour observed in the presence of strong scattering [7] , [18] , [19] . In general, Anderson localization is a statistical problem and the localization happens only strictly when averaged over many elements of a statistically identical ensemble. However, the large transverse scattering results in a strong self-averaging behaviour where the localized beam radius of each element of the ensemble is nearly equal to the average localized beam radius; therefore, the s.d. is small. Further details on the self-averaging property of highly scattering disordered fibres can be found in ref. 9 . The image transport quality is also independent of the polarization as shown in Supplementary Fig. 3 . The polarization of the output light was tested and was confirmed to retain its linear polarization with an extinction ratio of higher than 200. In ref. 9 , we noted that the results of the scalar wave equation were in excellent agreement with the full vectorial beam propagation method. Therefore, our experimental observations are consistent with the previous numerical simulations that polarization coupling is negligible in the p-ALOF image fibres for lengths under consideration in our experiments. Future efforts are focused on designing an air-glass disordered fibre with 50% air-hole fill-fraction, where the average size of the individual air-holes will be using numerical simulations optimized to obtain the minimum beam localization radius. We note that image transport has been investigated previously in random phase-separated glasses [23] , [24] . Unlike the p-ALOF, their reported structure lacks longitudinal invariance. Fabrication of an ideal air-glass disordered fibre is very challenging using the stack-and-draw techniques, considering that 100,000 or more elements must be used and the airholes must remain open after the draw. It may be possible to achieve this using a lower number of sites and by restacking/redrawing to obtain the required submicron resolution of the disorder. It may also be possible to use porous glass such as that reported in ref. 21 , albeit with a higher air-hole fill-fraction of nearly 50%. Future efforts will also include revisiting image transport in random phase-separated glasses and its relationship to transverse Anderson localization. Fabrication of the fibre A total of 40,000 pieces of PMMA and 40,000 pieces of PS fibres were randomly mixed; each fibre was 8 inches long with an approximate diameter of 200 μm. The mixture was fused together and redrawn to a fibre with a nearly square profile with an approximate side width of 250-μm. While some of the original randomly mixed fibres might have crossed over each other during the assembly and redraw process, the large redraw ratio guarantees that the refractive index profile remains relatively unchanged along the fibres in our experiments. The image fibres used for comparison with p-ALOF are from Fujikura (FIGH-10-350S and FIGH-10-500N) and are distributed by Myriad Fiber Imaging Technology, Incorporated. Experiments For imaging, we chose fibre samples of nearly 5 cm long and imaged a section of 1951 U.S. Air Force resolution test target (R1DS1N from Thorlabs) by directly butt-coupling the test target to the polished input end of the p-ALOF. The test target was directly illuminated by a diode laser at the wavelength of 405 nm, by a He-Ne at the wavelength of 633 nm, or by white light. The near-field output was imaged using 40 × and 60 × objectives onto a lensed CCD camera. Numerical simulations The images were propagated along the fibre by numerically solving the wave propagation equation described in ref. 9 . The illuminated image ‘UWM’ and number ‘6’ were created using the GIMP image editor and used as the input. The disordered refractive index profile was created by randomly assigning the refractive indexes of n 1 and n 2 to the different sites. The sites are square with the side width of 0.9-μm. Assessment of the image quality The most legitimate approach for determining the quality of an image that is viewed by a human eye is the subjective evaluation. However, subjective evaluation can be time consuming, expensive and impractical. Objective image quality assessment is used to closely approximate the subjective perception. Objective measures such as the mean squared error (MSE) and the peak signal to noise ratio (PSNR) [25] , [26] are developed for automatic evaluation of perceived images. MSE is the most widely used and simplest signal quality/fidelity measure [27] . It is computed by averaging the squared error between the pixel intensities of distorted and reference images where M and N are the horizontal and vertical pixel counts of the two images, X and Y , that are being compared. In the field of image processing, MSE is usually mapped to a peak signal to noise ratio (PSNR) that takes into account the dynamic range ( L ) of pixel intensities Despite the simplicity and clear physical meaning of MSE/PSNR, their quality assessment is not a good representation of the visually perceived quality and may result in large errors in quality assessment [25] . A highly effective method in the assessment of image quality is the structural similarity index (SSIM) that is developed based on the assumption that human visual system is greatly adapted for extracting structural information [25] . In SSIM, the quality of the transported images are compared with the distortion-free initial images that are launched into the fibres, by correlating the local pixel intensity patterns in different regions of the two images. The source of distortion in the transported images in the multicore image fibres studied here are the pixelation and coupling of light to adjacent cores. SSIM is used to compare the local image patches x and y from the same locations of the two images [27] . A simplified form of SSIM index is calculated using where μ x and μ y are local sample means of x and y , σ x and σ y are local sample s.d. of x and y , and σ xy is the cross correlation of samples x and y after subtracting their mean. C 1 and C 2 are positive numbers to stabilize the SSIM in cases of near zero mean, s.d. or cross correlation. C 1 and C 2 are defined as ( K 1 L ) 2 and ( K 2 L ) 2 where L is the dynamic range of the pixel intensities and K 1 <<1, K 2 <<1. To compare the quality of the transport images in the disordered optical fibres with the periodic imaging fibres, the quality of the transported images in both fibres are determined by mean structural similarity index (MSSIM). The MSSIM index is calculated by averaging the SSIM index where N is the number of local patches of the image and x j and y j are the image contents at the j th patch. How to cite this article: Karbasi, S. et al. Image transport through a disordered optical fibre mediated by transverse Anderson localization. Nat. Commun. 5:3362 doi: 10.1038/ncomms4362 (2014).